Ligand binding and aggregation of pathogenic SOD1 Mutations in the gene encoding Cu/Zn superoxide dismutase-1 cause amyotrophic lateral sclerosis. Superoxide dismutase-1 mutations decrease protein stability and promote aggregation. The mutant monomer is thought to be an intermediate in the pathway from the superoxide dismutase-1 dimer to aggregate. Here we find that the monomeric copper-apo, zinc-holo protein is structurally perturbed and the apo-protein aggregates without reattainment of the monomer–dimer equilibrium. Intervention to stabilize the superoxide dismutase-1 dimer and inhibit aggregation is regarded as a potential therapeutic strategy. We describe protein–ligand interactions for two compounds, Isoproterenol and 5-fluorouridine, highlighted as superoxide dismutase-1 stabilizers. We find both compounds interact with superoxide dismutase-1 at a key region identified at the core of the superoxide dismutase-1 fibrillar aggregates, β-barrel loop II–strand 3, rather than the proposed dimer interface site. This illustrates the need for direct structural observations when developing compounds for protein-targeted therapeutics. Amyotrophic lateral sclerosis (ALS) is a fatal human neuropathy characterized by death of the upper and lower motor neurons, leading to muscle atrophy and paralysis [1] . It is inexorably progressive with 70–80% of patients dying within 5 years of the onset of symptoms [2] . The first genetic factor to be unambiguously linked to ALS was the superoxide dismutase-1 (SOD1) encoding gene found on chromosome 21 at location q22.1 (ref. 3 ). Over 160 ALS-related mutations have now been discovered and an affected individual’s life expectancy after initial onset of symptoms is defined, to a large extent, by the mutation [4] , [5] , [6] . These mutations are diverse in nature and include amino acid deletion [7] and insertion [8] , deletion of base pairs in the 3′-untranslated region [9] , premature truncation [10] and amino acid substitution [3] . The mechanism of mutant SOD1 toxicity remains unclear. However, SOD1-containing inclusions are observed in cases of SOD1-related ALS, implicating SOD1 self-association as the pathogenic switch [11] , [12] . Familial ALS-associated mutations increase SOD1 aggregation propensity and predominantly reduce protein stability in vitro [13] , [14] , [15] . Although individually these characteristics do not affect the disease phenotype directly [15] , a synergistic interaction between aggregation propensity and protein stability strongly influences patient survival time after onset of symptoms [16] . Stabilization of the SOD1 dimer has been shown to increase the protein’s thermostability, prevent monomerization and inhibit aggregation [17] , [18] . The hypothesis that dimer destabilization promotes monomer formation, which in turn form high molecular weight inclusions, has directed attention towards stabilization of the dimer interface as a method for therapeutic intervention [19] , [20] . A large group of compounds have been described that have a putative capacity for binding SOD1 in a hydrophobic cavity created by Val7–Gly147–Val148 in the dimerization region [21] , [22] . Although several of this cohort have been shown to have potent aggregation inhibition activity, none have been validated by direct observation in situ . In 2004 we presented solution and crystal structures of A4V SOD1 and found there is significant and possibly pathogenic structural perturbation observable when the protein is present in solution [23] . In this study we provide evidence gained by small-angle X-ray scattering and in vitro aggregation experiments that the A4V SOD1 monomer is similarly structurally disturbed, destabilized and aggregation prone. However, we find the aggregation propensity of monomeric A4V SOD1 is lower than that of the dimer. Second, we contest the claim that a group of compounds designed to bind the dimer interface site [21] , [22] can inhibit SOD1 aggregation. We substantiate this by observation of SOD1 aggregation with Isoproterenol and 5-fluorouridine (5-FUrd), both of which have been reported to strongly inhibit dimer loss. Finally, we describe a ligand-binding site on the surface of the SOD1 β-barrel in a region important for SOD1 self-association, and characterize its interaction with a class of compounds that includes the catecholamine neurotransmitters. These observations have implications with regard to the mechanism of SOD1 pathogenicity and development of therapeutic agents. Structural perturbation of the A4V SOD1 monomer The combination of traditional small-angle scattering instrumentation and size exclusion chromatography (SEC-SAXS) has opened the way for the study of complex protein systems that are constituted by two or more species in solution [24] , [25] . Although dimeric at high concentrations, A4V SOD1 exists in a monomer–dimer equilibrium at low concentrations [17] . This presented us with the opportunity to observe the structure of the SOD1 monomer, a potential intermediate in the disease process [19] , [26] , for the severest and most prevalent of SOD1 mutants [27] . 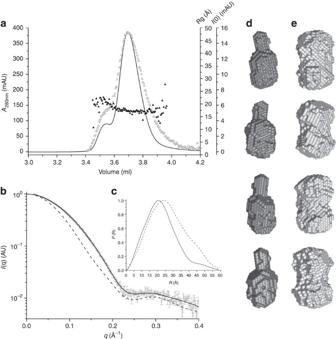Figure 1: The structure of monomeric recombinant A4V SOD1 determined by small-angle X-ray scattering. (a) A single size-exclusion chromatogram (see Methods) of monomeric recombinant Cu-apo, Zn-holo A4V SOD1 with radius of gyration (Rg; triangle) and forward scattering intensity (circle) plotted together with absorbance at 280 nm (line). (b) X-ray scattering profile of monomeric A4V SOD1 (solid line with experimental error derived from radial averaging of scattering frames in light gray) compared with the profile of dimeric wild-type SOD1 (dashed line). (c) Distance distribution function of monomeric A4V (solid line) and dimeric wtSOD1 (dashed line) (ref.60). (d) Space-filling model of monomeric A4V SOD1 and (e) wild-type dimeric SOD1. Figure 1a shows the size-exclusion chromatogram of Cu-apo, Zn-holo A4V SOD1 with small-angle scattering parameters plotted together with absorbance at 280 nm. The dimer and monomer species are visible at 3.53 and 3.7 ml, respectively, in both the A 280 nm and I (0) plots. Using SEC-SAXS, the radius of gyration (Rg) and maximum intraparticle dimension of dimeric wild-type SOD1 were 20.6±0.3 Å and 61 Å, in comparison with 21.4 Å and 74 Å for dimeric A4V. The A4V monomer is smaller with a radius of gyration (Rg) 17.05±0.3 Å and deduced molecular mass 15.6 kDa [28] , which equate well with the hydrodynamic radius and molecular mass of monomeric wild-type SOD1 determined by dynamic light scattering (19.4 Å and 17 kDa) [29] . The X-ray scattering profiles of the Cu-apo, Zn-holo A4V monomer and Cu-apo, Zn-holo dimeric wild-type SOD1 are similar with a characteristic minimum at 2.5 Å −1 . The distance distribution functions indicate proteins of approximately equal maximum dimension ( Fig. 1b respectively). This result is unexpected given the A4V monomer is half the molecular mass of the wild-type dimer and occurs owing to a single protrusion from the main body of the monomer ( Fig. 1d compared with e). This extended conformation is also observed in the dimeric A4V form [23] , indicating this structural disturbance is independent of oligomeric state. Figure 1: The structure of monomeric recombinant A4V SOD1 determined by small-angle X-ray scattering. ( a ) A single size-exclusion chromatogram (see Methods) of monomeric recombinant Cu-apo, Zn-holo A4V SOD1 with radius of gyration (Rg; triangle) and forward scattering intensity (circle) plotted together with absorbance at 280 nm (line). ( b ) X-ray scattering profile of monomeric A4V SOD1 (solid line with experimental error derived from radial averaging of scattering frames in light gray) compared with the profile of dimeric wild-type SOD1 (dashed line). ( c ) Distance distribution function of monomeric A4V (solid line) and dimeric wtSOD1 (dashed line) (ref. 60 ). ( d ) Space-filling model of monomeric A4V SOD1 and ( e ) wild-type dimeric SOD1. Full size image Monomeric apo-A4V SOD1 readily aggregates Dimeric and reduced apo monomeric A4V SOD1 have been shown to accumulate in an heterogeneous collection of high molecular weight soluble aggregates that increase in diameter as the incubation period increases [14] , [15] , [17] . 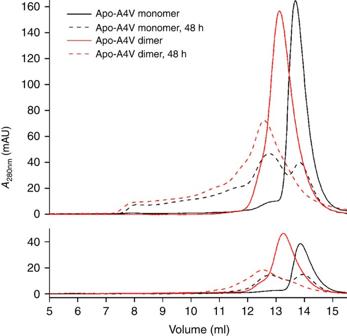Figure 2: Aggregation of monomeric and dimeric apo-A4V SOD1. Apo-A4V monomer and dimer size-exclusion chromatography elution profile obtained before and after 48 h incubation at 37°C. Upper panel shows protein at 100 μM and lower panel shows 25 μM. In each case, a single elution is measured by absorption at 280 nm. Figure 2 shows a comparison of the aggregation potential of monomeric and dimeric apo-A4V SOD1. Dimeric apo-A4V eluted from the SEC column at 13.1 ml. After 48 h, the dimer peak is almost completely absent and the majority of protein has moved to higher molecular weight species that elute with a peak at 12.6 ml. In contrast, monomeric A4V eluted at 13.7 ml and appears to aggregate more slowly. At concentrations that mimic the upper (100 μM) and lower (25 μM) bounds of intracellular SOD1 (ref. 29 ), 20 and 40% of the starting material remains as the monomer after 48 h. Aggregating protein accumulates in a species that elutes at 12.6 ml. It is interesting to note that in the metal apo form, both the monomer and dimer proceed to high molecular weight species, bypassing observable reattainment of the monomer–dimer equilibrium. This is the case at both high and low concentrations. Figure 2: Aggregation of monomeric and dimeric apo-A4V SOD1. Apo-A4V monomer and dimer size-exclusion chromatography elution profile obtained before and after 48 h incubation at 37 ° C. Upper panel shows protein at 100 μM and lower panel shows 25 μM. In each case, a single elution is measured by absorption at 280 nm. Full size image Putative SOD1 stabilizers do not inhibit aggregation Using an in silico screening approach, Lansbury and co-workers [21] , [22] identified a diverse array of chemical structures, which inhibited aggregation of A4V SOD1 in vitro . These compounds were postulated to bind a hydrophobic pocket created by opposing residues Val7, Gly147 and Val148 at the dimer interface. This was thought to stabilize the SOD1 dimer, and inhibit monomerization and slow aggregation. 5-FUrd, Isoproterenol and norepinephrine were found to inhibit SOD1 aggregation to such an extent that ~90% of the SOD1 dimer remained after a 48-h incubation in comparison with 40% if the compounds were not present [22] . To investigate the effect these compounds have on the aggregation of SOD1, the aggregation assay of Nowak et al . [22] was replicated using 25 and 100 μM monomeric and dimeric A4V SOD1. Two compound concentrations, a 1:3 and 1:30 molar excess of ligand, were used to ensure consistency and attempt to provide a sufficiency of bound ligand, respectively. Identical experiments were also performed with I113T SOD1, because aggregation has been well characterized for this mutant and has been proven inhibitable in vitro by licensed drug compounds [30] , [31] . 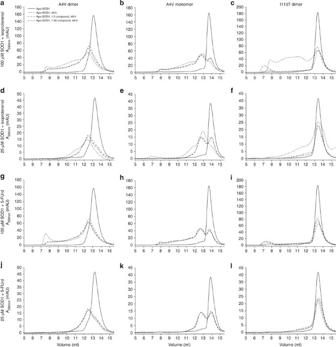Figure 3: Aggregation of apo-A4V and apo-I113T SOD1 in the presence of Isoproterenol and 5-FUrd. Size-exclusion chromatograms of apo-SOD1 with Isoproterenol and 5-FUrd after 48 h incubation at 37 °C compared with similarly treated protein without ligand and the fresh protein used as starting material for aggregation experiments measured at 280 nm. (a) 100 μM dimeric A4V SOD1 with 300 μM and 3 mM Isoproterenol. (b) 100 μM monomeric A4V SOD1 with 300 μM and 3 mM Isoproterenol. (c) 100 μM dimeric I113T SOD1 with 300 μM and 3 mM Isoproterenol. (d) 25 μM dimeric A4V SOD1 with 75 and 750 μM Isoproterenol. (e) 25 μM monomeric A4V SOD1 with 75 and 750 μM Isoproterenol. (f) 25 μM monomeric I113T SOD1 with 75 and 750 μM Isoproterenol. (g) 100 μM dimeric A4V SOD1 with 300 μM and 3 mM 5-FUrd. (h) 100 μM monomeric A4V SOD1 with 300 μM and 3 mM 5-FUrd. (i) 100 μM dimeric I113T SOD1 with 300 μM and 3 mM 5-FUrd. (j) 25 μM dimeric A4V SOD1 with 75 and 750 μM 5-FUrd. (k) 25 μM monomeric A4V SOD1 with 75 and 750 μM 5-FUrd. (l) 25 μM monomeric I113T SOD1 with 75 and 750 μM 5-FUrd. Each line is representative of a single chromatography run; however, figures showing similar chromatograms resulting from the average of triplicate separations of I113T with both 5-FUrd and Isoproterenol can be found inSupplementary Figs S1–S4. Figure 3 shows the size exclusion chromatograms for aggregated SOD1 in the presence of Isoproterenol and 5-FUrd. At 25 μM dimeric A4V and 75 μM compound ( Fig. 3d ), there is no inhibition of either dimer loss or accumulation of higher molecular weight species when compared with the control. This result is directly contradictory to the work of Nowak et al . [22] and is also seen at higher protein concentrations ( Fig. 3a ). Indeed, the chromatograms of SOD1 with 5-FUrd are almost indistinguishable from the controls at any of the concentrations assayed ( Fig. 3g–l and Supplementary Figs. S1–2 ) and are highly repeatable ( Supplementary Figs S1 and S2 ). Isoproterenol concentrations of 750 μM or 3 mM cause an increase in 280-nm absorbance over a region corresponding to high molecular weight species (7–13 ml; Fig. 3a–f and Supplementary Figs S3 and S4 ). Chromatography of 3 mM Isoproterenol after incubation without SOD1 indicates this compound spontaneously forms high molecular weight species ( Supplementary Fig. S5 ). This may relate to oxidation of the catechol alcohols and formation of melanin-like macromolecules, but these products do not elute concurrently with monomeric, dimeric or aggregated SOD1. In the case of A4V SOD1, there is a slight reduction in prevalence of the dimeric or monomeric starting material when compared with the control and low Isoproterenol concentration (75 and 300 μM) (Fig. 3a, b, d and e). These observations suggest high Isoproterenol concentrations may promote SOD1 oligomerization or the ligand is becoming incorporated into growing SOD1 aggregates causing an increase in 280 nm absorption. Figure 3: Aggregation of apo-A4V and apo-I113T SOD1 in the presence of Isoproterenol and 5-FUrd. Size-exclusion chromatograms of apo-SOD1 with Isoproterenol and 5-FUrd after 48 h incubation at 37 °C compared with similarly treated protein without ligand and the fresh protein used as starting material for aggregation experiments measured at 280 nm. ( a ) 100 μM dimeric A4V SOD1 with 300 μM and 3 mM Isoproterenol. ( b ) 100 μM monomeric A4V SOD1 with 300 μM and 3 mM Isoproterenol. ( c ) 100 μM dimeric I113T SOD1 with 300 μM and 3 mM Isoproterenol. ( d ) 25 μM dimeric A4V SOD1 with 75 and 750 μM Isoproterenol. ( e ) 25 μM monomeric A4V SOD1 with 75 and 750 μM Isoproterenol. ( f ) 25 μM monomeric I113T SOD1 with 75 and 750 μM Isoproterenol. ( g ) 100 μM dimeric A4V SOD1 with 300 μM and 3 mM 5-FUrd. ( h ) 100 μM monomeric A4V SOD1 with 300 μM and 3 mM 5-FUrd. ( i ) 100 μM dimeric I113T SOD1 with 300 μM and 3 mM 5-FUrd. ( j ) 25 μM dimeric A4V SOD1 with 75 and 750 μM 5-FUrd. ( k ) 25 μM monomeric A4V SOD1 with 75 and 750 μM 5-FUrd. ( l ) 25 μM monomeric I113T SOD1 with 75 and 750 μM 5-FUrd. Each line is representative of a single chromatography run; however, figures showing similar chromatograms resulting from the average of triplicate separations of I113T with both 5-FUrd and Isoproterenol can be found in Supplementary Figs S1–S4 . Full size image The instability of mutant SOD1 in comparison with the wild-type enzyme is well documented [14] , [15] , [32] , and stabilization of the protein is regarded as a viable strategy for drug development [18] . Isoproterenol and 5-FUrd were not assayed for a protective effect against chemically induced SOD1 denaturation by Nowak et al . [22] ; however, Lansbury and co-workers have used this method extensively to complement in silico docking and in vitro aggregation experiments [21] , [22] . 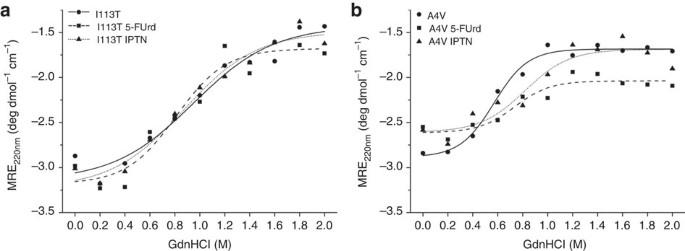Figure 4: Guanidine-induced unfolding of apo-I113T and apo-A4V SOD1 in the presence of Isoproterenol and 5-FUrd. (a) Apo-dimeric I113T unfolding in GdnHCl at 0.2 M concentration intervals with Isoproterenol or 5-FUrd monitored by ellipticity at 220 nm. The mid-point of the unfolding transition is found at 0.95, 0.87 and 0.81 M GdnHCl. (b) Apo-dimeric A4V unfolding in GdnHCl at 0.2-M concentration intervals with Isoproterenol or 5-FUrd monitored by ellipticity at 220 nm with unfolding transitions at 0.57, 0.81 and 0.73 M GdnHCl. In each case, unfolding is monitored by a single circular dichroism measurement. Figure 4 shows the guanidine hydrochloride (GdnHCl)-induced unfolding of I113T and dimeric A4V SOD1 in the presence of these two compounds. The unfolding transition shown is monitored using circular dichroism spectroscopy at 220 nm, which is typical for β-sheet-rich proteins [33] ; however, measurements at 230, 218, 215, 212, 210 and 208 nm indicated identical transitions. At low guanidine concentration (<2 M) apo-SOD1 is known to unfold [34] , and this is replicated here for both apo-I113T and apo-A4V with unfolding transitions at 0.81 and 0.57 M GdnHCl, respectively. This transition is not significantly shifted by the presence of a fourfold molar excess of Isoproterenol or 5-FUrd. Figure 4: Guanidine-induced unfolding of apo-I113T and apo-A4V SOD1 in the presence of Isoproterenol and 5-FUrd. ( a ) Apo-dimeric I113T unfolding in GdnHCl at 0.2 M concentration intervals with Isoproterenol or 5-FUrd monitored by ellipticity at 220 nm. The mid-point of the unfolding transition is found at 0.95, 0.87 and 0.81 M GdnHCl. ( b ) Apo-dimeric A4V unfolding in GdnHCl at 0.2-M concentration intervals with Isoproterenol or 5-FUrd monitored by ellipticity at 220 nm with unfolding transitions at 0.57, 0.81 and 0.73 M GdnHCl. In each case, unfolding is monitored by a single circular dichroism measurement. Full size image Putative SOD1 stabilizers do not bind at the dimer interface The structures of Isoproterenol and 5-FUrd-bound SOD1 were determined by single-crystal X-ray diffraction. The dimer interface mutant I113T grown in space group P2 1 with a single dimer in the asymmetric unit was used for initial crystallographic screening. This mutation was one of the first SOD1 mutations implicated in familial ALS (fALS) [3] , and is one of the most common SOD1 gene mutations. This particular crystal form regularly diffracts to atomic resolution, which aids ligand identification. To validate the binding site and determine if the interaction was an artefact of crystal packing, the compounds were observed in crystals of I113T SOD1 in the C222 1 space group with five dimers in the asymmetric unit. Finally, binding was confirmed in wild-type SOD1, as well as L38V and H48Q variants. Together with I113T, this group is a good representation of the full spectrum of SOD1 mutants. 5-FUrd is a fluorinated analogue of uridine monophosphate (UMP), but lacks the phosphate group at the 5′-position. On the basis of our previous investigations [35] , it would be expected to bind at the UMP-binding site between the zinc and electrostatic loops; however, 5-FUrd binding at Trp32 is the only observable interaction (4A7S, Fig. 5a–c , Supplementary Figs S6 and S10 , and Table 1 ). The fluorouracil group engages in aromatic stacking with Trp32, and the side chain of Ser98 acts as a hydrogen bond donor to the fluorouracil carbonyl adjacent to fluorine. In this instance, the indole of Trp32 displays two conformations. The ribose group shows significantly lower occupancy, as it is free to rotate about the anomeric C–N bond and projects away from the binding site into solvent. Although the reason for the switch in binding site between UMP and 5-FUrd is not fully clear, it is reasonable to suggest that although Trp32 is the preferred site, the highly polar nature of the phosphate present in UMP confers a destabilizing effect that precludes its binding there. 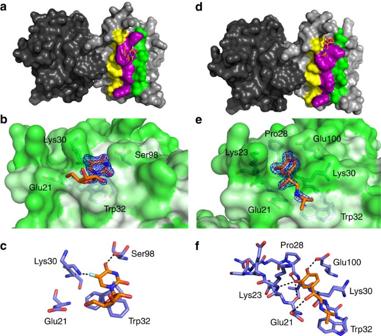Figure 5: 5-FUrd and Isoproterenol bound to I113T SOD1. (a) 5-FUrd with respect to the SOD1 dimer (4A7S) in grey and light grey; strands 2, 3 and 6 of the SOD1 β-barrel are coloured yellow, purple and green, respectively. (b) 2Fo-Fc electron density map of 5-FUrd contoured at 1σ at the Trp32-binding site with the SOD1 surface coloured by amino acid hydrophobicity. (c) Hydrogen bonding between I113T SOD1 and 5-FUrd shown with black dashed line. (d) Isoproterenol with respect to the SOD1 dimer (4A7T) coloured as ina. (e) 2Fo-Fc electron density map of Isoproterenol contoured at 1σ at the Trp32-binding site coloured as above. Little electron density is seen around the Isoproterenol tail; however, atoms in the catechol have an average B factor of 24.9 Å2and compare well with those of the Glu21 and Glu100 side chain carboxylates (average 23.0 Å2), indicating similar occupancy. (f) Hydrogen bonding between I113T SOD1 and Isoproterenol shown with black dashed line. Omit maps of both 5-FUrd and Isoproterenol bound to I113T SOD1 can be found inSupplementary Fig. S10. Figure 5: 5-FUrd and Isoproterenol bound to I113T SOD1. ( a ) 5-FUrd with respect to the SOD1 dimer (4A7S) in grey and light grey; strands 2, 3 and 6 of the SOD1 β-barrel are coloured yellow, purple and green, respectively. ( b ) 2Fo-Fc electron density map of 5-FUrd contoured at 1σ at the Trp32-binding site with the SOD1 surface coloured by amino acid hydrophobicity. ( c ) Hydrogen bonding between I113T SOD1 and 5-FUrd shown with black dashed line. ( d ) Isoproterenol with respect to the SOD1 dimer (4A7T) coloured as in a . ( e ) 2Fo-Fc electron density map of Isoproterenol contoured at 1σ at the Trp32-binding site coloured as above. Little electron density is seen around the Isoproterenol tail; however, atoms in the catechol have an average B factor of 24.9 Å 2 and compare well with those of the Glu21 and Glu100 side chain carboxylates (average 23.0 Å 2 ), indicating similar occupancy. ( f ) Hydrogen bonding between I113T SOD1 and Isoproterenol shown with black dashed line. Omit maps of both 5-FUrd and Isoproterenol bound to I113T SOD1 can be found in Supplementary Fig. S10 . Full size image Table 1 Crystallographic data collection and refinement statistics. Full size table The bradycardia therapeutic isoproterenol (isoprenaline) is appealing due to its ‘rule of three’ compliance, which makes it a promising candidate for a fragment-based drug-discovery approach [36] . This compound is also interesting, as it has been shown to dramatically decrease SOD1 transcription in rats [37] . The high-resolution structure of cocrystals with I113T SOD1 (4A7T) displayed no indications of binding at the dimer interface site, but Isoproterenol was found in a hydrophilic pocket created by SOD1 loop II ( Fig. 5d–f , Supplementary Figs S7, S10, S11 and Table 1 ). The backbone carbonyls of Glu21 and Pro28 along with the backbone amide NH of Gln22 interact with one of the catechol hydroxyl groups. The other forms a hydrogen bond to the side chain of Glu100. The amino alcohol side chain may also interact with the Glu21 side-chain carboxylate. The isopropyl group resides above Trp32, possibly taking advantage of a hydrophobic interaction with the side-chain indole; however, its occupancy is lower than the rest of the molecule indicative of a degree of flexibility. In the absence of ligand, the side chain of Lys30 has a significant degree of conformational freedom. However, in the presence of Isoproterenol it is forced to move towards Ser98. Isoproterenol is structurally related to the neurotransmitters dopamine and epinephrine. 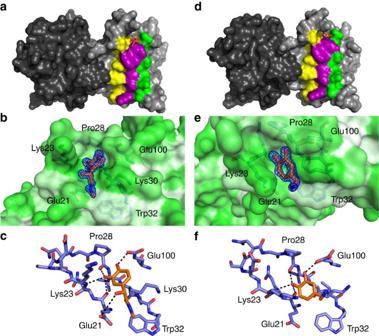Figure 6: Epinephrine and dopamine bound to I113T SOD1. (a) Epinephrine with respect to the SOD1 dimer (4A7U) in grey and light grey; strands 2, 3 and 6 of the SOD1 β-barrel are coloured yellow, purple and green, respectively. (b) 2Fo-Fc electron density map of epinephrine contoured at 1σ at the Trp32-binding site with the SOD1 surface coloured by amino acid hydrophobicity. Average B factor of the catechol head is 16.6 Å2in comparison with 21.7 Å2for the Glu21 and Glu100 side chain carboxylates. (c) Hydrogen bonding between I113T SOD1 and epinephrine shown with black dashed line. (d) Dopamine with respect to the SOD1 dimer (4A7U) coloured as above. (e) 2Fo-Fc electron density map of dopamine contoured at 1σ at the Trp32-binding site coloured as above. Average B factor of the catechol head is 25.0 Å2compared with 32.8 Å2for the Glu21 and Glu100 carboxylates when refined at full occupancy. (f) Hydrogen bonding between I113T SOD1 and dopamine shown with black dashed line. Omit maps of epinephrine and dopamine bound to I113T SOD1 can be found inSupplementary Fig. S10. In view of the findings above, X-ray crystal structures of both compounds bound to I113T SOD1 were subsequently obtained (4A7U and 4A7V, respectively, Figure 6 , Supplementary Figs. S8, S9 and S10 , and Table 1 ). Both were clearly visible in the same binding site as Isoproterenol and with comparable conformations, although the plane of the catechol head group is rotated in the case of dopamine. In this case, no hydrogen-bonding interactions can take place with Glu100, because of the absence of a tail hydroxyl. Figure 6: Epinephrine and dopamine bound to I113T SOD1. ( a ) Epinephrine with respect to the SOD1 dimer (4A7U) in grey and light grey; strands 2, 3 and 6 of the SOD1 β-barrel are coloured yellow, purple and green, respectively. ( b ) 2Fo-Fc electron density map of epinephrine contoured at 1σ at the Trp32-binding site with the SOD1 surface coloured by amino acid hydrophobicity. Average B factor of the catechol head is 16.6 Å 2 in comparison with 21.7 Å 2 for the Glu21 and Glu100 side chain carboxylates. ( c ) Hydrogen bonding between I113T SOD1 and epinephrine shown with black dashed line. ( d ) Dopamine with respect to the SOD1 dimer (4A7U) coloured as above. ( e ) 2Fo-Fc electron density map of dopamine contoured at 1σ at the Trp32-binding site coloured as above. Average B factor of the catechol head is 25.0 Å 2 compared with 32.8 Å 2 for the Glu21 and Glu100 carboxylates when refined at full occupancy. ( f ) Hydrogen bonding between I113T SOD1 and dopamine shown with black dashed line. Omit maps of epinephrine and dopamine bound to I113T SOD1 can be found in Supplementary Fig. S10 . Full size image Familial ALS SOD1 mutants are predominantly detrimental to protein stability and universally promote aggregation [15] . Wild-type and fALS-associated mutant SOD1 proteins have been found to be aggregation prone in vitro , particularly when demetallated [30] , [38] . Apo-I113T SOD1, for example, undergoes a gradual but progressive disappearance of the dimeric form concomitant with evolution of higher molecular weight species when analysed by size-exclusion chromatography after incubation at physiologically relevant concentration, pH and temperature, without the necessity of agitation [30] . Here we have observed the aggregation of an homogenous monomeric apo-SOD1 species. We find that, similar to the dimeric species [17] , monomeric apo-A4V is prone to aggregation, but the rate is slower. Surprisingly, under these conditions there is no substantial reattainment of a monomer–dimer equilibrium even at low concentration. These observations are in agreement with data implicating monomeric SOD1 in the aggregation process [19] , [29] , but do not support a pivotal role. One would expect the monomer to aggregate faster than the dimer if monomerization were a rate-limiting step. Conversely, faster aggregation by the dimer may be a reflection of the fact that no monomer–dimer transition must occur first, or that the dimer is more readily incorporated into growing oligomers. Monomeric SOD1 has previously been observed by dynamic light-scattering, circular dichroism and tryptophan fluorescence [19] , [29] . These experiments indicated a protein with similar size parameters to those described here, but with little or no conformational rearrangement. The low-resolution SAXS model of the zinc-loaded A4V monomer is not, as expected, roughly spherical, but has a projection that extends the maximum particle dimension equal to that of the wild-type SOD1 dimer. This protuberance is reflected in the SAXS-derived solution structure of the A4V dimer [23] , but the low-resolution nature of SAXS does not allow us to unambiguously assign this mass to a particular region of the SOD1 polypeptide. However, given the absence of a circular dichroism spectral shift in the monomeric as opposed to dimeric protein, this structural disturbance must arise without modification of any optically active structural feature. An obvious choice in respect of this would be untethering of one of the flexible loops, which are thought to provide protection to the central SOD1 β-barrel. Structural perturbation of the electrostatic loop, in particular, has been observed in a wide range of SOD1 mutants and is predicted by molecular dynamics simulation of the apo-A4V monomer [39] , [40] . In addition to β-barrel deprotection, this structural disturbance could be detrimental to copper retention or loading by the SOD1 copper chaperone. In this last case, the structurally important intra-subunit disulphide may also be affected. Stabilization of the SOD1 dimer interface has emerged as a potential strategy for the development of a therapeutic agent for SOD1-related fALS [18] , [20] , [21] , [22] . Isoproterenol and 5-FUrd have previously been shown to inhibit aggregation of A4V SOD1 in vitro and also demonstrate selectivity for SOD1 in blood plasma [22] . Site-directed mutagenesis experiments and the use of in silico screening had predicted their binding to the dimer interface and provided a rationale for their activity. However, our X-ray crystallographic studies clearly show that 5-FUrd binds at Trp32 and Isoproterenol binds at a previously unobserved site close to, but distinct from, the Trp32-binding site. The interactions described have been tested against wild-type and a range of representative SOD1 mutants (I113T, L38V and H48Q) and found to be highly repeatable. In no case is there evidence of ligand binding at the Val7–Gly147–Val148 site as predicted by in silico studies [21] , [22] . Familial ALS mutations are found throughout the full length of the SOD1 polypeptide; however, the β-strand-3 region is suspiciously free and is the longest stretch without a known mutation. One could speculate this is because the region is critically important for modulation of the self-association characteristic and, in support of this, it has been shown to exhibit local unfolding in ALS SOD1 mutants [41] . Oxidation of the Trp32 indole side chain also results in formation of covalent aggregations of SOD1, and a W32S mutation in a fALS SOD1-mutant protein abolishes propagation of SOD1 aggregation [42] , [43] , [44] . Furthermore, three key regions of SOD1 are found in the core of protein fibrillar aggregates, one of which spans Ala1–Lys30 and another Asp90–His120 (ref. 45 ). With the exception of Trp32, these regions encompass all the strand 2–loop II–strand 3 residues identified in the course of this investigation. Further evidence for the importance of the binding sites presented here was identified by analysis of the amino acid sequence of SOD1, using the Waltz amyloid-prediction algorithm [46] . This highlights the region Val14–Gln22 as a potential amylogenic region [47] and is in agreement with one of the regions identified experimentally by Furukawa et al . [45] In view of these points, it is disappointing to find that SOD1 resistance to chaotrope-induced unfolding is unchanged in the presence of Isoproterenol or 5-FUrd and the previously reported inhibition of aggregation could not be confirmed. Norepinephrine was also highlighted as a SOD1 aggregation inhibitor [22] . Given the discovery that epinephrine binds at the loop II site, we assayed this compound for aggregation inhibition and found no effect. The lack of reliable in vitro assays to use as a yard stick in SOD1 therapeutics development may be hampering targeted drug development. Affinity data is an important part of protein–ligand interaction characterization and is essential if more specific, tighter binding compounds are to be recognized. Despite our best efforts, an abundance of protein and highly soluble ligands, we were unable to acquire this data using isothermal titration calorimetry or 1H NMR line broadening, indicating that dissociation constants for Isoproterenol and 5-FUrd at the sites described are in the mid-low millimolar range. With this binding affinity we suggest that the three molar excess of ligand used in the original work [22] is insufficient to drive the compound into the binding site; therefore, any effect in terms of aggregation inhibition could never be attributed to site-specific binding at the loop II region or the Val7–Gly147–Val148 site. Since SOD1 was unambiguously linked to ALS in 1993 (ref. 3 ), it has posed numerous challenges in the continuing search for the molecular cause of its pathogenicity and it is often still enigmatic and mystifying. From a fragment-based drug-discovery perspective, it is a difficult protein to tackle, due in large part to the absence of conspicuous binding sites. The Val7–Gly147–Val148 dimerization region site and the active site are the only obvious candidates upon which to dock small molecules. The loop II and Trp32-binding sites presented here, and in our previous work [35] , [48] , are unusual in that they are highly solvent exposed, but they harbour the only validated SOD1–ligand interactions outside the active site. Given their location, they may prove invaluable as we move to inhibit aberrant SOD1 self-association and are good starting point for computational optimization. This case study highlights that the overwhelming advantages of direct observation of drug leads at their target sites. In-silico modelling is well adapted to generate many compounds with potential binding activity against a target and has a critical role in developing those compounds into therapeutics. However, the gold standard is validation of that binding by visualization in situ . With this information, structure activity relationship models can be rationalized with understanding of the compounds’ molecular interactions with the target. As a result, optimization is likely a much more efficient process and the drug-discovery pipeline shorter. Recombinant SOD1 production and crystallization Recombinant untagged hSOD1 I113T, L38V and wild-type proteins were produced by expression in E. coli BL21 (DE3) cells driven by a pET303C-SOD1 plasmid and purified by ammonium sulphate cut followed by hydrophobic interaction chromatography. Expression from this system yields and a 153 amino acid SOD1 protein. Crystals in the P2 1 space group were grown at 20 °C in 100 mM NaOAc pH 4.75, 150 mM NaCl using 2 M (NH 4 ) 2 SO 4 as precipitant by the hanging-drop vapour diffusion method from a pre-existing seed. I113T SOD1 crystals in the C222 1 space group grew spontaneously at 20 °C in 100 mM Tris-HCl pH 8, 150 mM NaCl and 2.0 M (NH 4 ) 2 SO 4 . All crystallization proceeded from stock SOD1 solutions of 5–10 mg ml −1 . Recombinant SOD1 proteins used in SEC aggregation assays, chemical unfolding and SAXS experiments were produced as above; however, purification was by ion-exchange chromatography on diethylaminoethanol sepharose followed by gel filtration on a Superdex 200 16/60 column in Tris-buffered saline pH 7.4. The SOD1 A4V variant was produced according to Ray et al . [17] Monomeric or dimeric protein was purified by SEC on a Superdex 200 16/60 column. Where necessary, apo-SOD1 was produced according to McCord and Fridovich [49] . In all cases, SOD1 concentration was determined by ultraviolet spectroscopy using a monomeric molar extinction coefficient at 280 nm of 5,500 M −1 cm −1 . Ligand soaking and X-ray crystallography Crystals grown in the P2 1 space group were soaked with compounds (50 mM) dissolved in 2.5 M (NH 4 ) 2 SO 4 , 150 mM NaCl, 100 mM NaOAc pH 4.75 solution for 2 h at 20 °C. Crystals grown at pH 8 in the C222 1 space group were soaked in compounds (50 mM) dissolved in 2.5 M (NH 4 ) 2 SO 4 , 150 mM NaCl, 100 mM Tris-HCl pH 8. X-ray crystallographic data sets were collected at the Diamond Light Source stations I02 an I03, Oxford, UK, and at the Soleil station Proxima 1, Saint-Aubin, France. Reflection data were integrated and scaled using HKL2000 (ref. 50 ), XDS [51] , or iMosflm [52] and Scala [53] . Cycles of model building and refinement proceeded using REFMAC5 [54] and COOT [55] . Crystallographic data collection, scaling and refinement statistics for I113T SOD1 in the P2 1 space group are presented in Table 1 . SOD1 aggregation Aggregation of SOD1 was performed according to Nowak et al . [22] Apo-SOD1 at 25 or 100 μM and compound at 1:3 or 1:30 concentration were mixed in each assay in a 350 μl volume and incubated for 15 min before addition of 5 mM EDTA, wherein they were incubated at 37 °C for 48 h. Samples (300 μl) were analysed by ultraviolet light absorption at 280 nm on a Superose-12 column, using an ÄKTA purifier 100 with flow rate 0.5 ml min −1 . SOD1 chemical unfolding SOD1 unfolding in the presence of ligands was performed according to Nowak et al . [22] Isoproterenol or 5-FUrd were added to 25 μM apo-SOD1 and incubated at room temperature for 15 min before addition of GdnHCl. The GdnHCl concentration was confirmed by refractive index and samples from 0 to 4 M at 0.2 M step intervals were prepared. Unfolding was left to proceed for 12 h at room temperature before measurement. Far ultraviolet circular dichroism spectroscopy (200–250 nm) was performed on a Jasco J-810 spectropolarimeter with path length 0.5 mm, bandwidth 2 nm, step resolution 0.1 nm, scan rate 50 nm min −1 and response time 2 s at 25 °C. Measurements are an average of five readings. Protein unfolding was observed by fitting a two-state model to readings taken at 220 nm. Small-angle X-ray scattering Monomeric copper-apo, zinc-holo A4V SOD1 was determined to be homogenous by SDS–PAGE and its was identity confirmed by peptide mass fingerprinting. It was analysed using the combined HPLC–SAXS setup at beamline SWING [24] as follows: 100 μl of 350 μM protein was loaded onto an Agilent Bio SEC-5 HPLC column, using an Agilent 1200 HPLC at 200 μl min −1 at 10 °C. Small-angle scattering parameters were calculated for a series of 250 exposures (starting at 3 ml and lasting 1,000 ms separated by 500 ms dead time) taken as the protein eluted with 100 frames taken before the column void volume for buffer subtraction. The incident beam had wavelength 1.03 Å and the sample-detector distance was 1.782 m. One hundred buffer frames were averaged and subtracted from ten frames corresponding to an elution volume of 3.68–3.73 ml, which were then averaged to yield the scattering profile. A Guinier approximation was performed with Primus [56] , and the distance distribution function was calculated using q range up to 0.4 Å −1 with GNOM [57] . Twenty ab initio models were constructed using GASBOR [58] and were averaged with DAMAVER [59] . Accession codes : Atomic coordinates and structure factors for the crystal structures have been deposited in Protein Data Bank under accession numbers 4A7S, 4A7T, 4A7U and 4A7V , 4A7T , 4A7U and 4A7V . How to cite this article : Wright, G. S. A. et al . Ligand binding and aggregation of pathogenic SOD1. Nat. Commun. 4:1758 doi: 10.1038/ncomms2750 (2013).